Microscopic response to inhomogeneous deformations in curvilinear coordinates A mechanical deformation of a continuum can be expressed as a generalized coordinate transformation of space. Consequently, the equations of electrostatics in deformable media must satisfy covariance requirements with respect to such transformations, a problem that has long been addressed in the context of general relativity. Here we show how these ideas can be incorporated into the framework of density-functional perturbation theory, providing access to the microscopic charge density and electrostatic potential response to an arbitrary deformation field. We demonstrate the power of our approach by deriving, in full generality, the surface contributions to the flexoelectric response of a finite object, a topic that has recently been a matter of controversy. The breakdown of translational periodicity produces consequences that might seem highly paradoxical at first sight: for example, the macroscopic bulk polarization does not always correspond to the physical surface charge. The electrical response of a material to deformations has been an increasingly popular topic in condensed matter during the past decades. Such an interest has been fuelled both by the intriguing fundamental physics that governs electromechanical couplings and by the technological importance of signal conversion, for example, in sensors, actuators or energy harvesters. Until very recently, the word ‘electromechanical’ was almost exclusively referred to piezoelectricity and electrostriction, respectively, the linear and quadratic coupling between the polarization ( P ) and a uniform strain. In the past few years the advent of flexoelectricity (that is, the linear response of P to a strain gradient) has brought to the field an entirely new range of challenges and opportunities, both in device design and in fundamental science [1] , [2] , [3] , [4] , [5] . Although the attention of the research community has traditionally been focused on the macroscopic electromechanical response of solids, there are increasingly good reasons to investigate what happens, during a deformation, at a smaller length scale. This is certainly true for a number of emerging device concepts (for example, foldable inorganic light-emitting diodes [6] or energy harvesters based on semiconductor nanowires [7] ) whose operation critically depends on how the (spatially resolved) electrostatic potential responds to a strain field. More generally, miniaturization trends in electronics have reached a stage where device performance can no longer be understood in terms of the bulk properties of the constituents [8] , [9] , calling for design rules that treat the active element as a whole quantum-mechanical object. In the case of flexoelectricity, such a paradigm shift seems unavoidable: here the contribution of the sample boundaries is believed [10] , [11] to be much more profound than, for example, in the piezoelectric case, to the point that the very nature of flexoelectricity as a bulk effect is currently under debate [10] , [12] . Finally, inhomogeneous deformations produce intriguing physical consequences in two-dimensional nanostructures, for example, geometric fields [13] , electronic flexoelectricity [14] and a ‘pseudomagnetic’ quantum Hall effect [15] . To develop realistic models of the aforementioned phenomena, one clearly needs to go beyond the macroscopic picture and focus on local response functions, that is, understand how the electron charge, electric fields and polarization individually respond to the deformation at the microscopic level. First-principles electronic-structure calculations, particularly in the framework of density-functional perturbation theory (DFPT), appear ideally suited to answering such questions with unbiased accuracy. Macroscopic deformations, however, have traditionally required special precautions to be tractable within DFPT, as they typically change the boundary conditions of the Hamiltonian. [16] Viable methodologies exist to calculate, in full generality, the response of a periodic system to a uniform strain [17] . Extending these techniques to the case of a strain gradient perturbation, is, however, far from trivial. Here, due to the inherent breakdown of translational periodicity, even representing the response functions on an appropriate regular grid appears problematic. Here we address the above methodological issues by reformulating DFPT [16] on a curvilinear coordinate system. This allows us to derive, via long-wave expansion of quantities that can be readily calculated by means of publicly available codes, the microscopic charge density and polarization response to an arbitrary deformation field. We show how a general-relativistic revision of Maxwell equations (and of the relevant scalar and vector quantities) is instrumental to achieving this goal. Application of this formalism to the flexoelectric response of an unsupported slab demonstrates the existence of surface-dependent contributions that do not vanish in the thermodynamic limit, consistent with the phenomenological arguments of Tagantsev and Yurkov [11] . We further clarify the physical nature of such contributions, which can adopt the form of a surface dipole or charge, depending on the type of strain gradient perturbation. In the Supplementary Notes 1, 2 and 3 we illustrate these findings by means of analytical and numerical examples. Preliminaries We shall base our formalism on the lattice-dynamical theory of ref. 18 , where the response of a periodic crystal to deformations was derived from a long-wave analysis of acoustic phonons. The fact that the present work is primarily (but not exclusively) aimed at systems that are finite along at least one spatial direction is not a major drawback here: any low-dimensional object (for example, a slab) can be recast as a periodic crystal by means of the supercell method (see Fig. 1 ). Consider a crystal lattice spanned by the real-space vectors R l , and by N basis atoms located at τ κ ( κ =1,…, N ) within the primitive cell. 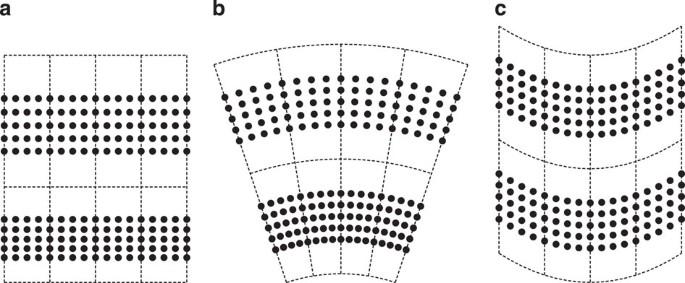Figure 1: Slab supercell subjected to a macroscopic strain gradient. The three main types of strain gradients producing a dipole moment normal to the surfaces are shown: longitudinal (a), transverse (b) and shear (c). The supercell boundaries are shown as dashed lines, the slabs are schematically represented as arrays of black circles. Suppose that each atom, identified by the cell index l and by the sublattice index κ , undergoes a small displacement of the type Figure 1: Slab supercell subjected to a macroscopic strain gradient. The three main types of strain gradients producing a dipole moment normal to the surfaces are shown: longitudinal ( a ), transverse ( b ) and shear ( c ). The supercell boundaries are shown as dashed lines, the slabs are schematically represented as arrays of black circles. Full size image that is, a ‘frozen-ion’ acoustic phonon, with a κ -independent eigenvector U β . (To avoid overburdening the notation, for the time being we shall restrict our analysis to frozen-ion deformations; ionic relaxations will be dealt with in a later section. Note that the expression ‘frozen-ion’ is used here with the same meaning as in the study by Hong and Vanderbilt [19] , that is, it should not be confused with the rigid-ion model of Tagantsev [10] .) The electronic response to such a perturbation can be expressed as a phase times a cell-periodic function [18] , where f is either the induced charge density, ρ , or one of the three components of the microscopic polarization vector, P α . With the precaution of adequately screening the macroscopic electric fields, in the limit of small q (long wavelength), the cell-periodic part of the response can be Taylor-expanded in powers of q around the Γ point. The microscopic charge density and polarization responses are then, to second order in the wavevector q (ref. 18 ), where both and are invariant under β ↔ γ exchange. In ref. 18 , we showed that the macroscopic (frozen-ion) piezoelectric and flexoelectric tensors can be written, respectively, in terms of the cell averages of and . In the following sections we shall focus more specifically on the microscopic response functions. Coordinate transformations Our goal is to recast Equation (3) and Equation (4) in a such a way that they express the response of the system to ‘proper’ measures of the local deformation only. These are the symmetric strain tensor, ε βγ , and the strain gradient tensor, η β , γλ (ref. 18 ). To achieve this goal, the first difficulty we need to face is understanding how to deal with the zero-order terms in the q -expansions, respectively, and . These correspond to rigid translations of the whole lattice and can be expressed in terms of the unperturbed charge density, ρ ( r ), and originate from the fact that we have derived our response functions in the fixed reference frame of the unperturbed crystal. Although this is the most natural way of describing a phonon perturbation, in the present context of macroscopic deformations such a choice is problematic as it introduces a dependence of the response functions on the absolute position (and rotation angle) of the crystal at rest. To overcome this obstacle, we propose to express all the response functions in the curvilinear coordinate system, r , that is defined by the following mapping to the original Cartesian frame, r ′, In r , the atoms do not move from their lattice positions: only the local metric [17] and its gradients are ‘aware’ of the deformation; therefore, both and disappear by construction. The central question to be solved then is how the basic laws of electrostatics are modified by a generalized coordinate transformation such as Equation (6). An elegant solution to this problem was recently proposed in the context of metamaterials [20] , where general-relativistic transformation of coordinates led to substantial breakthroughs in the design of advanced optical devices (for example, perfect lenses or invisibility cloaks) [21] , [22] . Given an arbitrary coordinate transformation r ′= r ′( r 1 , r 2 , r 3 ), one first needs to redefine the basic electrostatic quantities as follows [21] , [22] , where h αβ is the ‘deformation gradient’, and E ( r ) is the electric field. Then, based on , and , the microscopic Maxwell equations can be directly written in the curved system [21] , [22] , that is, Gauss’s law retains essentially the same form as in the flat Cartesian space, except for the replacement of the vacuum permittivity with the tensor ( g = h · h T is the metric of the deformation; indicates the nabla operator in the curvilinear reference.) As is the gradient of the electrostatic potential, V (the latter is an invariant scalar), the above equations yield the microscopic V ( r ) from the knowledge of the charge or polarization field. (Alternatively, one can arrive at Equation (11) by observing that, in a curvilinear space, the Poisson equation of electrostatics must be rewritten as that is, the Laplacian must be replaced with the Laplace–Beltrami operator, where g =det( g )=det 2 ( h ). Then, by defining , , and , one immediately recovers Equation (11).) Interestingly, the above prescriptions coincide with the definition of the reduced electrical variables, which were introduced by Stengel et al. [23] to facilitate the treatment of coupled electromechanical problems in periodic crystals. (If we consider the linear transformation between reduced lattice coordinates and Cartesian coordinates, then h αβ is the β component of the translation vector α . It is easy to verify that the symbols and p α of ref. 23 correspond to and , respectively.) More generally, such a revised formulation was shown to fix many undesirable ambiguities of the ‘standard’ theory of deformable dielectric media [24] , [25] . Linear response We shall now apply the above prescriptions to the coordinate transformation Equation (6). Equation (8) has no effect on P in the linear regime (the polarization of the crystal at rest can be assumed to be identically zero). Conversely, Equation (9) introduces an additional contribution to via the determinant of h γβ ( r )= δ γβ + iq γ U β e i q · r , of the form iq γ δ βγ ρ ( r ). Recall that the deformation gradient h corresponds to the unsymmetrized stress tensor and that the type-I strain gradient tensor is η β , γλ ( r )=∂ 2 r ′ β /∂ r γ ∂ r λ =− q γ q λ U β e i q · r . Then we can write where we have replaced the unsymmetrized strain tensor h γβ with the symmetrized one, ε βγ , thanks to the invariance of both and with respect to β ↔ γ exchange [18] . This is a central result of this work, expressing (in a fully translationally and rotationally invariant form) the basic electrostatic fields in the curvilinear system as a function of quantities that are defined (and can be readily calculated) in the standard Cartesian reference. It is easy to verify that the fundamental relationship holds, confirming the internal consistency of our theory. We still need the electric field and potential, which we shall discuss hereafter. By expanding Equation (11) to linear order in the perturbation, we obtain where is minus the (curvilinear) gradient of the induced electrostatic potential, Δ V . The additional ‘metric’ contribution to the polarization, coming from the linearization of , reads ( is the electric field in the unperturbed system.) Note that does not contribute to the macroscopic flexoelectric response of a periodic system ( averages to zero over the supercell) but does contribute to the response of a finite object, as we shall illustrate shortly. Equation (15) specifies modulo an r -independent integration constant, whose value is fixed by the electrical boundary conditions (EBC) of the problem. The electronic response functions are typically defined (and calculated [18] ) by assuming short-circuit ( ) conditions, however, any conceivable EBC choice can be recovered if the charge–density (and/or polarization) linear response to a macroscopic electric field is known. (Note that is first-order in the perturbation, and therefore its contribution to the electronic response functions is only due to the microscopic dielectric properties of the unperturbed system.) For example, in the case of the polarization one can write where is the microscopic P response to an applied field along β [26] . The contribution of this term can be readily incorporated into P (2) , and therefore Equation (14) remains valid in arbitrary EBC. This concludes our derivations, good for computing the microscopic charge, polarization and electric field response of an arbitrary crystal (or finite object) to an inhomogeneous ‘frozen-ion’ deformation. In the following section we shall demonstrate the above formalism by addressing the problem of the surface flexoelectric response. Surface flexoelectric response Consider for simplicity a symmetrically terminated slab of a cubic material, whose surfaces (which we assume parallel to the yz plane) are insulating and have the highest symmetry compatible with the underlying bulk lattice (for example, a (100)-oriented slab of a rocksalt insulator). Unless specified otherwise, we set the electrical boundary conditions in such a way that the macroscopic electric field deep in the interior of the slab always vanishes. We shall consider the three independent types of strain gradient deformations (see Fig. 1 ) that induce a dipole moment normal to the surface plane: longitudinal ( ε xx , x ), transverse (or bending, ε yy , x ) and shear ( ε xy , y ). The former two cases are qualitatively similar: the strain increases along the direction normal to the surface, so in-plane periodicity is preserved. (In the transverse case this observation is far from trivial—it implies that the y Cartesian coordinate is folded to a torus geometry and acquires the meaning of an angle.) By rewriting Equation (14) in type-II form (recall the relationship [18] between type-I and type-II strain gradient tensors, η α , βγ = ε αβ , γ + ε γα , β — ε βγ , α ), we obtain (only the x component of P has a non-zero contribution because of symmetry) where and are the planar and macroscopic averages (given a function f , planar averaging consists in taking its mean value over the surface cell area S , ; macroscopic averaging [27] , [28] , [29] consists in convoluting f ( x ) with a filtering function g ( x ), whose width is of the order of the interatomic spacing) of and of respectively. ( is the type-II counterpart [18] of P (2) .) An illustration of the polarization field induced by a transversal deformation (the longitudinal case is qualitatively similar) of the slab is shown in Fig. 2a,c . 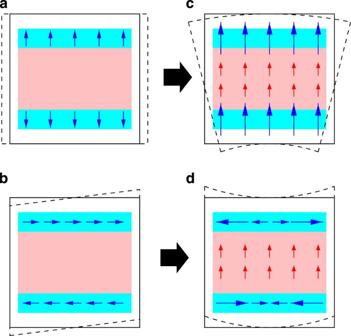Figure 2: Polarization fields induced by a macroscopic deformation. Left panels (a,b) illustrate a uniformly strained slab; right panels (c,d) represent the same slab subjected to uniform strain gradients. Top (a,c) are transverse deformations (the situation is qualitatively similar in the longitudinal case, not shown), bottom (b,d) are shear patterns. The surface regions and corresponding polarization fields are indicated by light blue shading and blue arrows, respectively. Red arrows on a pink background refer to the bulk region. The continuous and dashed black frames indicate the type of deformation in each case. Figure 2: Polarization fields induced by a macroscopic deformation. Left panels ( a , b ) illustrate a uniformly strained slab; right panels ( c , d ) represent the same slab subjected to uniform strain gradients. Top ( a , c ) are transverse deformations (the situation is qualitatively similar in the longitudinal case, not shown), bottom ( b , d ) are shear patterns. The surface regions and corresponding polarization fields are indicated by light blue shading and blue arrows, respectively. Red arrows on a pink background refer to the bulk region. The continuous and dashed black frames indicate the type of deformation in each case. Full size image We are interested in the total dipole density per unit volume induced by the strain gradient deformation, where L is the slab thickness. In the limit of a macroscopically thick slab ( L →∞), the result is where is the bulk frozen-ion flexoelectric tensor [18] and the surface contribution is given by (We indicate the centre of the vacuum region as x =+∞; we use a bar symbol to indicate frozen-ion quantities, consistent with the notation of ref. 18 .) Note that vanishes at the centre of the slab ( x =0), as we assumed that the bulk material is not piezoelectric and the slab is symmetrically terminated. Conversely, near the surface this function is generally non-zero due to the broken-symmetry environment. Hence, is a surface-specific property that always yields a finite, thickness-independent contribution to the overall flexoelectric coefficient of the slab. By construction, is the linear variation in the surface dipole moment induced by a uniform strain, ε αα . To obtain the total surface contribution to the flexoelectric response of the slab, , we need to take into account, in addition to , the metric contribution to the first-order electric field . We obtain where is the surface electrostatic potential offset (also called ‘lineup’ term [29] ) of the slab at rest. It is straightforward to verify that is the linear variation in the surface electrostatic lineup induced by a uniform strain, consistent with the arguments of Hong and Vanderbilt [19] . The physical interpretation of this result is best illustrated by adopting open-circuit (OC) boundary conditions, as shown schematically in Fig. 3a,b . The unperturbed system is a symmetrical quantum well with no dipole. Upon deformation, a uniform electric field, , builds up in the bulk region ( is the high-frequency dielectric constant of the bulk material). At the same time, two collinear dipoles (both equal to ) are induced at the opposite surfaces, producing (together with the metric part discussed above) an antisymmetric contribution to the potential profile. The sum of these three contributions, sketched in Fig. 3a , yields the potential profile shown in Fig. 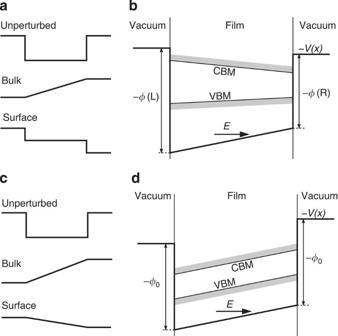Figure 3: Schematic band diagram of a deformed slab. We assume open-circuit boundary conditions, that is, the electric field must vanish outside the slab boundaries. Panelsa,billustrate the effect of a longitudinal or transverse strain gradient; panelsc,dcorrespond to a shear one. Inaandcthe individual contributions to the electrostatic potential are shown. The diagramsbanddshow the overall result, and also indicate the location of the valence (VBM) and conduction (CBM) band edges. The electrostatic potential,V(x), and the left (φ(L)), right (φ(R)) and unperturbed (φ0) lineup terms are all reported with a minus sign, as the band diagram refers to electrons (with negative charge). The electric field is indicated byEand an arrow pointing right. 3b , corresponding to a total potential offset, V OC , of Figure 3: Schematic band diagram of a deformed slab. We assume open-circuit boundary conditions, that is, the electric field must vanish outside the slab boundaries. Panels a , b illustrate the effect of a longitudinal or transverse strain gradient; panels c , d correspond to a shear one. In a and c the individual contributions to the electrostatic potential are shown. The diagrams b and d show the overall result, and also indicate the location of the valence (VBM) and conduction (CBM) band edges. The electrostatic potential, V ( x ), and the left ( φ (L)), right ( φ (R)) and unperturbed ( φ 0 ) lineup terms are all reported with a minus sign, as the band diagram refers to electrons (with negative charge). The electric field is indicated by E and an arrow pointing right. Full size image (The constant K accounts for size effects occurring at finite values of L , see Supplementary Note 2 for further details.) Once the electrostatic potential has been determined, the position of the band edges can be located by adding to − V ( x ) the usual bulk band-structure term [29] , which is analytic (that is, it depends only on the local strain at x ). This is fully consistent with the theory of absolute deformation potentials [30] , which we formally extend here to the transverse case of a bending deformation and to the treatment of the surface part. It is worth mentioning that the above conclusions could be equivalently obtained from an analysis of the charge density response. Although the latter (unlike the polarization response) does not lead to an obvious separation between bulk and surface effects, its use might be convenient in practical calculations. (An illustration of this point is provided in Supplementary Note 1 .) The counterpart of Equation (18) in the charge density case is (Here, again, we have performed the necessary planar and macroscopic averages and converted ρ (2) to type-II form.) By integrating one recovers , and from one can then extract all the relevant physical quantities. Interestingly, as we know already that surface effects in the longitudinal and transversal case can only contribute to the surface dipole (and not to the surface charge), this analysis gives us access to the bulk flexoelectric coefficient in terms of the surface charge–density response alone, This result can be especially uesful to calculate the transverse bulk coefficient ( x ≠α), which is difficult to access by means of the currently available implementations [19] , [31] . The case of the shear strain gradient ( ε xy , y ) is qualitatively different from those discussed above, in that the strain linearly increases parallel to the surface plane (along y here), rather than perpendicular. This implies that the polarization response is no longer periodic in plane; however, as we work under the assumption that the strain varies slowly compared with the interatomic spacings, we can still write it in terms of macroscopically averaged quantities, ( α can be either x or y ; both are, in principle, allowed.) The second term at the right-hand side of Equation (26) reduces (in the thermodynamic limit) to the bulk flexoelectric coefficient , and is zero by symmetry for α = y . Conversely, the other term vanishes for α = x : a uniform shear deformation of the slab does not affect the surface dipole (again, by symmetry). The α = y contribution does not vanish: is a transversal surface current induced by uniform shear ( Fig. 2b ). In a shear strain gradient, Equation (26), this transversal current increases linearly parallel to the surface ( Fig. 2d ), and thus produces a net surface density of bound charge, (Note that Equation (27) is similar in form to Equation (21), although the signs are opposite.) The resulting OC band diagram is illustrated in Fig. 2d . With respect to the previous (longitudinal or transverse) case the surface dipolar contribution is absent, and there are no band-structure contributions either (all bands are parallel). The surface effects manifest themselves in the internal field, which is, therefore, not a bulk property in the shear case (see Fig. 2c ). Note that the internal field is not only due to the ‘physical’ surface charge density Δ σ surf plus the bulk flexoelectric coefficient but also due to the ‘metric’ field , which acts like an additional surface charge density, We identify the sum of Equation (27) and Equation (28) as the surface flexoelectric coefficient in the shear case, . In Supplementary Note 1 we discuss an extreme case where Δ σ surf and Δ σ met exactly cancel, that is, there is a net surface charge but a vanishing , highlighting the importance of a consistent treatment of all contributions to the overall response. Atomic relaxations So far, for simplicity, we have not considered the possibility that the atoms may relax in a given deformation field. Lattice-mediated effects are obviously of utmost importance for a realistic description of flexoelectric phenomena. In the following section we shall demonstrate that the theory developed in this work can be easily adapted to incorporate such effects. In the long-wave limit, the atomic displacements associated with an acoustic phonon can be written, to second order in q , as [18] where κ is a sublattice index, and are the piezoelectric and flexoelectric (type-I) internal-strain tensors and ω is the frequency. By following the same line of reasoning as we did for the frozen-ion polarization and charge density response, it is easy to show that Γ and N describe the microscopic lattice response to the deformation in the curvilinear coordinate system specified by r ′ β = r β + U β e i q · r − iωt , (Here R lκ = R l + τ κ .) It is equally easy to show that Equation (13) and Equation (14) still hold, provided that one replaces the frozen-ion charge density and polarization response functions with their relaxed-ion counterparts. For example, in the case of the polarization response, one has (The symbols in the previous equations differ from those introduced in Equation (4) by the presence of the sublattice index, κ . They are defined by operating Equation (1) only on atoms κ . The sublattice sums of the former quantities yield the latter ones. Note that the cell integral of corresponds to the Born dynamical charge tensor, . Further details are reported in ref. 18 .) Finally, to adequately treat the effect of the electrical boundary conditions it is also necessary to revise Equation (17) by including ionic relaxations in the electric field response function, . This formally extends the microscopic linear-response theory of the present work to the relaxed-ion case, for an insulating crystal of arbitrary symmetry and composition. Hereafter, we shall describe the impact of atomic relaxations on the flexoelectric response of the free-standing film that we discussed in the previous section. Consider, as above, a slab supercell (see Fig. 1 ), where the vacuum layers are thick enough to avoid any interaction between the repeated images of the film. We shall again analyse the three types of strain gradient deformation that are schematically illustrated in Fig. 1 . In the context of ionic relaxations, it is of primary importance to understand whether the flexoelectric response is of static or dynamic nature. The known dependence of the type-I internal-strain tensor , as well as of its type-II counterpart, on the atomic masses [18] indicates that the effect is, in general, dynamic. Recall, however, that such mass dependence scales [18] with the macroscopic elastic tensor of the periodic crystal, . Now, the relevant components of (longitudinal xx,xx , transverse and shear ) all vanish in a slab supercell due to the absence of interactions across the vacuum layer. Thus, in the specific case of the slab supercell, the corresponding components of both N and L are independent of masses, and therefore unsensitive to the static or dynamic nature of the strain gradient perturbation. Based on this result, we can now proceed to discussing each individual case without ambiguities. It is not difficult to see that a longitudinal strain gradient produces no electrical dipole and, in fact, leaves the slab unperturbed. Indeed, given the absence of slab–slab interactions, a longitudinal acoustic phonon with propagation direction normal to the surface is a zero-frequency mode at any q , where each repeated image of the slab moves as a rigid object. Note that the response functions of Equation (31), Equation (32) and Equation (33) do not vanish—the slab remains unperturbed in the Cartesian frame, and not in the curvilinear frame to which and refer. Such response functions are, however, trivial (for example, , with X l κ =( R l κ ) x ), and their interest is only limited to the purpose of switching between different coordinate systems; we shall see an example shortly where such an operation is actually quite convenient. A transversal strain gradient (corresponding to a pure bending deformation) is physically more interesting than the longitudinal case. A straightforward application of Equation (31) leads to where we have expressed all the relevant tensors in type-II form. One can show that the piezoelectric internal-strain tensor can be written as where remains finite in the limit of large slab thicknesses; the contribution that is linear in X 0 κ is governed by the parameter which is related to the Poisson’s ratio of the bulk material. The ν -dependent term stems from elementary elasticity: as the surfaces are free to relax, the interior of the slab develops a macroscopic longitudinal strain ε xx =− νε yy in response to the perturbing transversal strain. (Similarly, a transversal strain gradient induces a longitudinal strain gradient, and their ratio is governed by the same constant of proportionality, ν .) To facilitate the analysis it is thus convenient to consider, rather than a pure transverse strain (or strain gradient), effective deformations of the type Note that the inclusion of the longitudinal components has no effect on the electrical response of the slab. This prescription is really just a coordinate transformation, whose purpose is to ensure that the macroscopic strain gradient of the supercell exactly matches the elastic state of the bulk material deep within the film. We have where . One can verify that both and tend to the corresponding bulk tensors far from the surfaces and that the surface-specific deviations are independent of slab thickness (provided that the slab is not too thin). Straightforward algebra leads to the induced electrostatic potential step on bending in open-circuit boundary conditions, where is the static bulk flexoelectric tensor, ∈ st is the static bulk dielectric constant, and is the variation in the surface potential offset induced by a uniform transversal strain after full ionic relaxation. (As above, K ′ is a surface-specific constant, irrelevant in the limit of large L .) This expression is formally identical to Equation (23), except for the replacement of the frozen-ion quantities with their relaxed-ion counterparts. In Supplementary Note 3 we provide a numerical example to illustrate the above results in a practical context. The third and last case of a shear strain gradient is relatively straightforward to analyse in light of the results presented so far. The induced atomic displacements read Regardless of the microscopic details of the slab, rotational invariance dictates that that is, under a uniform shear the slab rigidly rotates to accomodate the deformation of the supercell, without feeling any restoring force because the repeated images of the slab are decoupled. This implies that a shear strain gradient applied to a free slab inevitably produces a second strain gradient component, of the type −2 η y , xy . The overall effect is that of a negative transversal strain gradient, This means that, for a free-standing film, the shear case reduces exactly to the transversal one. The important conclusion is that flexoelectric effects in a free-standing film are governed by only one parameter, which is the radius of curvature, R , of the film (recall that ε yy , x =1/ R ) at the location where the induced potential is measured. All conceivable strain gradient deformations, either static or dynamic, are then described by one single flexoelectric coefficient, given by Equation (41). The above results have profound implications for the theoretical understanding of flexoelectric phenomena, and for the interpretation of the relevant experiments. In all the cases that we have explicitly considered, there are unavoidable surface contributions to the total dipole of a deformed slab, whose magnitudes increase linearly with the slab thickness. The relative importance of bulk and surface effects, therefore, is independent of thickness: both contributions persist in the limit of a macroscopically thick sample, and seem difficult to separate by purely electrical means. Note that such a difficulty is not just an experimental one: as a matter of principle, the very definition of the individual bulk and surface contributions is ambiguous [18] when taken separately. The two must go together, and the arbitrariness disappears only when they are summed up. This implies that the interpretation of recent experiments where flexoelectric properties of materials were measured (for example, Zubko et al. [3] and Ma and Cross [32] ) should be done with some caution, and the impact of the surface characteristics assessed in each case. From the theoretical point of view, first-principles calculations of flexoelectric properties that were reported to date [19] , [31] , [33] , [34] almost exclusively focused on bulk coefficients; it would be desirable in the future to gain quantitative insight on the degree of variability that the surface-dependent contribution entails. To give a more quantitative illustration of the above statements, we have applied the formalism developed in this work to two simplified toy models: a simple-cubic lattice of noninteracting closed-shell atoms ( Supplementary Note 1 ) and a two-dimensional lattice of atoms interacting with classical forces ( Supplementary Notes 2 and 3 ; the model parameters are reported in Supplementary Table S1 ). In both cases we consider a slab geometry subjected to the three types of strain gradient deformation discussed in this work ( Supplementary Fig. S1 ); either the frozen-ion ( Supplementary Note 1 and 2 ) or relaxed-ion ( Supplementary Note 3 ) response is computed. We find that, in all cases, surface effects can have a dramatic impact (that is, of the same order of magnitude as the bulk contribution) on the overall flexoelectric response of the slab. Moreover, the total electrostatic potential often results from the subtle cancellation of several different contributions ( Supplementary Fig. S2 ; Supplementary Tables S2 and S3 ), highlighting the crucial importance of all terms (including the metric part) for obtaining a correct physical answer. Although these results corroborate our conclusions, a full first-principles implementation of the present methodology would be highly desirable, in order to test these ideas on a realistic material. The surface contribution that we derive in this work can be directly linked to the ‘surface piezoelectricity’ that was recently discussed by Tagantsev and Yurkov [11] . Although Tagantsev and Yurkov [11] did recognize, based on phenomenological arguments, that such surface effect is comparable to the bulk contribution regardless of sample thickness, they did not, however, provide precise indications on its microscopic physical nature. The relevance of the surface potential offset was recognized by Hong and Vanderbilt [19] , although their work, being primarily focused on bulk properties, did not explore in depth the implications of this effect for the flexoelectric properties of a slab. The present work brings these results together into a unified and general linear-response theory, whose scopes are by no means limited to thin films but can be used to study an essentially endless variety of nanostructures and low-dimensional systems (for example, bent manifolds [13] , sp 2 -bonded crystals such as graphene [14] and boron nitride [35] , or semiconductor nanowires [7] ). Thus, the stage is set for attacking a wealth of curvature-related materials science problems with full ab initio power; applications to systems of technological and fundamental relevance are under way. How to cite this article: Stengel, M. Microscopic response to inhomogeneous deformations in curvilinear coordinates. Nat. Commun. 4:2693 doi: 10.1038/ncomms3693 (2013).